AmotL2 links VE-cadherin to contractile actin fibres necessary for aortic lumen expansion The assembly of individual endothelial cells into multicellular tubes is a complex morphogenetic event in vascular development. Extracellular matrix cues and cell–cell junctional communication are fundamental to tube formation. Together they determine the shape of endothelial cells and the tubular structures that they ultimately form. Little is known regarding how mechanical signals are transmitted between cells to control cell shape changes during morphogenesis. Here we provide evidence that the scaffold protein amotL2 is needed for aortic vessel lumen expansion. Using gene inactivation strategies in zebrafish, mouse and endothelial cell culture systems, we show that amotL2 associates to the VE-cadherin adhesion complex where it couples adherens junctions to contractile actin fibres. Inactivation of amotL2 dissociates VE-cadherin from cytoskeletal tensile forces that affect endothelial cell shape. We propose that the VE-cadherin/amotL2 complex is responsible for transmitting mechanical force between endothelial cells for the coordination of cellular morphogenesis consistent with aortic lumen expansion and function. The genesis of biological tubes is central to the physiology of glandular organs and the vascular circulatory network. In vertebrates, the primary axial blood vessels, the dorsal aorta (DA) and cardinal vein, are formed through vasculogenesis. During this process, individual mesodermal angioblasts migrate to the embryonic midline and differentiate into endothelial cells. Upon reaching their destination, endothelial cells elongate to form parallel cords followed by the formation of a central lumen allowing for the initiation of circulation [1] , [2] , [3] , [4] . Recent investigations have shed light on the molecular mechanisms of aortic lumen formation (reviewed in refs 3 , 5 , 6 ). Model systems recreating endothelial tubulogenesis in vitro have identified the cytoskeleton, apical–basal polarity as well as cell–cell adhesion components as being crucial for lumenization of tubes [7] . This has been further emphasized by studies of aortic lumen formation by genetic inactivation in mouse where modulators of the cytoskeleton (RASIP1), polarity (beta1 integrin and Par3) and cell–cell adhesions (VE-cadherin) all show luminal defects of the DA [8] , [9] , [10] , [11] . Aortic lumen expansion is synchronized with the onset of cardiac function, which suggests a tight coordination of these signalling pathways with flow-induced morphological changes of endothelial cells during vascular development. The de novo development of blood vessels in response to morphogenic gradients of growth factors such as VEGF has been extensively studied (reviewed in refs 1 , 12 , 13 , 14 , 15 ). Less is known about how endothelial cells perceive and transmit mechanical forces that modulate vessel shape and function. Extracellular forces are detected by endothelial cells via integrins in focal adhesions that form contact points that transfer tension from the extracellular matrix to the cytoskeleton [16] . Recent evidence has also shown that actomyosin contractility may be transmitted via adherens junctions [17] . Exogenous forces applied to cadherin have indicated a mechanical coupling between the cytoplasmic domains of cadherin and the actin cytoskeleton. Furthermore, in vitro measurements of force transmission have revealed that cell–cell contact-forming cells sustain endogenous forces that are directed towards the cell junctions [18] , [19] , [20] . VE-cadherin is a major component of endothelial adherens junctions. It regulates several aspects of endothelial biology including vascular integrity, permeability and blood vessel morphogenesis [21] . During embryonic vasculogenesis, VE-cadherin is essential for lumenization, and loss of VE-cadherin function resulted in endothelial apical–basal polarity and cytoskeletal defects [2] , [8] , [22] , [23] . VE-cadherin regulates the actin network since dynamic remodelling of adherens junctions is closely associated with the appearance of contractile actin fibres [24] . The actin-binding protein α-catenin is considered to be a dedicated mediator between cadherin and the actin cytoskeleton. However, this idea has been revised in favour of a more dynamic model where the α-catenin switch regulates a balance of linear versus branched actin cables depending on its association with ancillary proteins [25] . Although recent evidence indicates that VE-cadherin play an important role in force transmission, the molecular connection to the actin cytoskeleton remains obscure [26] . AmotL2 belongs to the Angiomotin (amot) family of membrane-associated scaffold proteins and contains an amino-terminal glutamine-rich domain coiled-coil repeats and a carboxy-terminal PDZ-binding domain, which together structurally define the Amot family [27] . Functional analyses of Amot and amotL1 in mouse and zebrafish have demonstrated specific roles in polarity in angiogenic tip cell migration and endothelial cell junction stability, respectively [28] , [29] , [30] . Amot coordinates cell migration and cellular shape by coupling RhoA activity to the leading edge and thereby affecting formation of actin fibres [31] . In this report, we have addressed how endothelial cells integrate mechanical forces via adherens junctions during the formation of the aortic lumen. We present data suggesting that the amotL2/VE-cadherin junctional complex is part of machinery translating junctional signals to actin cytoskeleton-driven cell shape changes, which are essential for aortic lumen expansion. AmotL2 expression in zebrafish endothelial cells The zebrafish has emerged as an important model system to analyse the complex development of the primary vessels, the DA and the posterior cardinal vein (PCV) and the expansion of the vascular network by angiogenic sprouting. In zebrafish, amotl2 is duplicated with paralogues on chromosomes 6 ( amotl2a ) and 2 ( amotl2b ) ( Supplementary Fig. 1a ). Endothelial expression of amotl2a and 2b was detected by quantitative PCR in fluorescence-activated cell sorting Tg(fli1a:EGFP) y1 cells from transgenic embryos where EGFP expression is driven by the fli1a endothelial specific promoter ( Supplementary Fig. 1b ). In addition, the amotl2a gene has previously been shown to be expressed in the DA, PCV and intersegmental vessels (ISVs) [32] . AmotL2a is required for DA lumen formation In order to determine whether amotl2 is required for vascular development, we individually targeted amotl2a and amotl2b functions in zebrafish using paralogue-specific morpholinos (MO). The effects on the vascular system were monitored using double transgenic embryos, where erythrocytes express dsRed ( Tg(gata1:dsRed) sd2 ) and the vascular endothelial network is visualized via EGFP ( Tg(kdrl:EGFP) s843 ). In agreement with the earlier results, we found that amotl2a depletion resulted in embryos with gastrulation defects [32] . However, at lower morpholino concentrations, amotl2a MO-injected embryos went through gastrulation properly, but exhibited pericardial oedema starting at 28 h post fertilization (h.p.f.) ( Fig. 1a ). Knockdown of amotl2b with morpholinos also resulted in pericardial oedema, but did not affect gastrulation ( Fig. 1a ). Confocal imaging of amotl2a and amotl2b morphant embryos revealed the establishment of both the major axial vessels, PCV and DA, as well as sprouting of ISVs and cranial vessels ( Fig. 1a,b and Supplementary Fig. 2a ). However, in morphant embryos, dsRed-positive erythrocytes accumulated in the areas of pericardial oedema whereas no circulating cells in the trunk vasculature could be detected ( Fig. 1a,b , Supplementary videos 1,2 ). Simultaneous knockdown of amotl2a and 2b paralogues, hereafter referred to as amotl2 MO, phenocopied the individual morphant phenotypes ( Fig. 1a,b ). Morpholino knockdown efficiency, phenotypic reproducibility and specificity were confirmed in control experiments ( Fig. 1c–e , Supplementary Fig. 1c,d,e ). 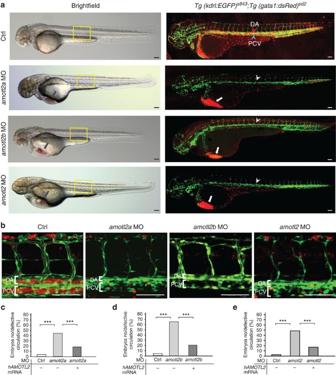Figure 1: AmotL2 depletion affects zebrafish circulation. (a) Brightfield (left) and fluorescent images (right) of 48 h.p.f. double transgenic embryos where red blood cells express dsRed (Tg(gata1:dsRed)sd2) and endothelial cells are visualized by EGFP (Tg(kdrl:EGFP)s843); control,amotl2a, amotl2b,andamotl2a/b(hereafter referred to asamotl2 MO)injected embryos (morphants).amotl2morphants show loss of trunk circulation (arrowhead) and peri-yolk oedema (arrow), even though they have beating hearts. DA and PCV are marked with red and blue arrowheads, respectively (top panel). Scale bar, 100 μm. (b) Magnified images (yellow box in a) show loss of dsRed-positive erythrocytes in the morphant ISVs and DA. DA morphogenesis is affected in amotL2 morphants, while the PCV is unaffected (brackets indicate vessel diameter). At 48 h.p.f., both the ISVs and dorsal anastomosing vessel were present, but lacked patent lumens. The lack of visible lumens in ISVs is due to the absence of blood flow in the aorta. Scale bar, 50 μm. (c–e) Rescue ofamotl2a(c),amotl2b(d) andamotl2 MO(e) defects by co-injection with full-length wild-type humanamotL2p100 mRNA demonstrating that the circulatory defects are specifically caused by loss ofamotl2function.n≥60 embryos per group, ***P≤0.001 as calculated by theλ2test. Figure 1: AmotL2 depletion affects zebrafish circulation. ( a ) Brightfield (left) and fluorescent images (right) of 48 h.p.f. double transgenic embryos where red blood cells express dsRed ( Tg(gata1:dsRed) sd2 ) and endothelial cells are visualized by EGFP ( Tg(kdrl:EGFP) s843 ); control, amotl2a, amotl2b, and amotl2a/b (hereafter referred to as amotl2 MO) injected embryos (morphants). amotl2 morphants show loss of trunk circulation (arrowhead) and peri-yolk oedema (arrow), even though they have beating hearts. DA and PCV are marked with red and blue arrowheads, respectively (top panel). Scale bar, 100 μm. ( b ) Magnified images (yellow box in a) show loss of dsRed-positive erythrocytes in the morphant ISVs and DA. DA morphogenesis is affected in amotL2 morphants, while the PCV is unaffected (brackets indicate vessel diameter). At 48 h.p.f., both the ISVs and dorsal anastomosing vessel were present, but lacked patent lumens. The lack of visible lumens in ISVs is due to the absence of blood flow in the aorta. Scale bar, 50 μm. ( c – e ) Rescue of amotl2a ( c ), amotl2b ( d ) and amotl2 MO ( e ) defects by co-injection with full-length wild-type human amotL2 p100 mRNA demonstrating that the circulatory defects are specifically caused by loss of amotl2 function. n ≥60 embryos per group, *** P ≤0.001 as calculated by the λ 2 test. Full size image In both the individual amotl2a and amotl2b knockdown embryos, and especially in the amotl2 MO double morphants, constrictions within the DA were observed ( Fig. 2a ). Lumen narrowing was invariably found along the length of the DA, but never in the PCV (95% aortic origin, 0% vein, 5% unknown, n =62) ( Fig. 2a ). DA lumen defects were not a secondary defect to the loss of blood circulation based on two observations. First, amotl2 morphants retained rhythmic heartbeat ( Supplementary videos 3, 4 ). Second, dorsal aortic lumen defects were not observed in silent heart / tnnt2 morphants, which lack heartbeat and vascular flow ( Supplementary Fig. 3a ) [33] . Accordingly, both amotl2a and amotl2b were required for proper DA morphogenesis. 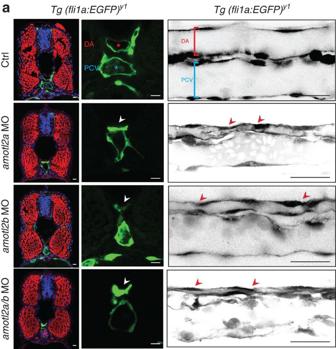Figure 2: DA lumen constrictions inamotl2MO morphants. (a) Transverse sections (left, thickness 200 μm) from 48 h.p.f.Tg(fli1a:EGFP)y1fish stained with phalloidin (red) to image F-actin and TO-PRO-3 iodide (blue) to label nuclei. In close up (mid panel), control embryos show a patent DA lumen (red asterisk) and a patent PCV lumen (blue asterisk). Scale bar, 10 μm. Luminal DA constrictions are present inamotl2a,amotl2bandamotl2MO morphants (arrowheads). The appearance of a midline aorta inamotl2MO indicated that midline directed migration was unaffected. Sagittal views (right) of the DA (red brackets show vessel diameter) and PCV (blue brackets show vessel diameter) in control andamotl2morphants.amotl2morphants show DA constrictions (red arrowheads) and reduced DA diameter. Scale bar, 50 μm. Figure 2: DA lumen constrictions in amotl2 MO morphants. ( a ) Transverse sections (left, thickness 200 μm) from 48 h.p.f. Tg(fli1a:EGFP) y1 fish stained with phalloidin (red) to image F-actin and TO-PRO-3 iodide (blue) to label nuclei. In close up (mid panel), control embryos show a patent DA lumen (red asterisk) and a patent PCV lumen (blue asterisk). Scale bar, 10 μm. Luminal DA constrictions are present in amotl2a , amotl2b and amotl2 MO morphants (arrowheads). The appearance of a midline aorta in amotl2 MO indicated that midline directed migration was unaffected. Sagittal views (right) of the DA (red brackets show vessel diameter) and PCV (blue brackets show vessel diameter) in control and amotl2 morphants. amotl2 morphants show DA constrictions (red arrowheads) and reduced DA diameter. Scale bar, 50 μm. Full size image AmotL2 is required for endothelial elongation The aortic lumen defects in amotl2 MO may have been caused by defective cell proliferation, cell morphogenesis or polarity. Cell counts showed no difference between the control and morphant aortic endothelium. We turned our attention to endothelial cell shape during aortic tube formation. By injecting a fli1a :mCherry containing plasmid into Tg(fli1a:EGFP) zebrafish embryos, individual aortic endothelial cells were mosaically labelled with mCherry. In zebrafish, aortic endothelia have a flattened and elongated morphology ( Fig. 3a ) [34] . The dimensions of individual mCherry-positive DA endothelial cells were quantified by calculating the length to width and the length to height ratios (bidirectional arrows, Fig. 3a ). Quantification of these morphometric ratios showed a significant defect in anteroposterior elongation in amotl2 -depleted embryos ( Fig. 3b,c ). These morphological changes could be restored by co-injection with human AMOTL2 messenger RNA (mRNA) ( Fig. 3a,b,c ). 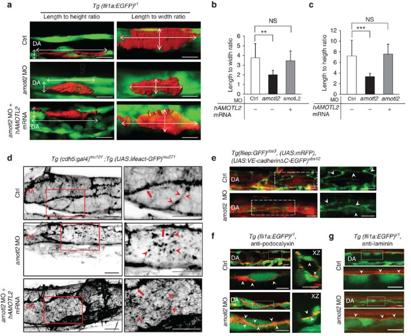Figure 3: Aortic endothelial cell shape and cytoskeletal defects inamotl2MO. (a) Sagittal (left) and dorsal (right) view of a mCherry-labelled DA endothelial cell of a 30 h.p.f. zebrafish embryo. Images show three-dimensional surface reconstruction of individual mCherry-expressing cells within the DA. Bidirectional arrows indicate the length and width dimensions. Inamotl2MO, DA endothelial cells show altered cell shape. These morphological changes as well as the lumen defect can be reversed by injection of a humanamotL2mRNA. Scale bar, 10 μm. (b) Quantification of length to width ratio in individual mCherry positive, control andamotl2MO aortic endothelial cells, as well asamotl2MO cells rescued by co-injection with humanamotL2mRNA (controln=18 cells,amotl2MOn=10 cells,amotl2MO+hAMOTL2mRNAn=11 cells, Ctrl versusamotL2MOP=0.011, Ctrl versusamotL2MO+hamotL2mRNAP=0.541. (c) Quantification of length to height ratio in individual mCherry positive, control andamotl2MO aortic endothelial cells (Ctrl versusamotL2MOP=0.0003, Ctrl versusamotL2MO+hamotL2mRNAP=0.722).P-values were calculated by student’st-test. Error bars indicate s.d. NS, non significant. (d) Endothelial actin cytoskeletal structure visualized in the dorsal aortic endothelia from living 48 h.p.f.Tg(cdh5:gal4)mu101;Tg(UAS:lifeact-GFP)mu271transgenic fish. Red boxes indicate magnified areas (right). Arrowheads show actin filaments present in the control, and punctuate actin in theamotl2MO. Arrows indicate cortical actin present in both control andamotl2MO embryos. By introducing humanamotL2mRNA, actin filaments could be restored (arrowheads). Scale bar 10 μm. (e) In controlTg(fliep:GFF)ubs3; (UAS:mRFP); (UAS:VE-cadherinΔC-EGFP)ubs12embryos (top), where VE-cadherin is tagged to EGFP, and endothelial cells labelled by mRFP, VE-cadherin enmarks cell–cell junctions. InamotL2MO embryos (bottom), VE-cadherin is still localized in between endothelia at sites of aortic constrictions. Boxed areas are magnified to the right, VE-cadherin–EGFP signal indicated with arrowheads. Scale bar 10 μm. (f) The apical-membrane sialomucin podocalyxin (arrowheads) is retained in apical membranes ofamotl2MO DA constrictions. ControlTg(fli1a:EGFP)y128 h.p.f. embryos (top) andamotl2MO (bottom). Boxed areas are magnified below. This is also visualized in the optical transverse section (XZ, right). Scale bar, 10 μm. (g) In controlTg(fli1a:EGFP)y128 h.p.f. embryos (top), anti-laminin staining is basal (arrowheads) and inamotl2MO, anti-laminin staining is unaffected (arrowheads, bottom). Scale bar, 10 μm. Figure 3: Aortic endothelial cell shape and cytoskeletal defects in amotl2 MO. ( a ) Sagittal (left) and dorsal (right) view of a mCherry-labelled DA endothelial cell of a 30 h.p.f. zebrafish embryo. Images show three-dimensional surface reconstruction of individual mCherry-expressing cells within the DA. Bidirectional arrows indicate the length and width dimensions. In amotl2 MO, DA endothelial cells show altered cell shape. These morphological changes as well as the lumen defect can be reversed by injection of a human amotL2 mRNA. Scale bar, 10 μm. ( b ) Quantification of length to width ratio in individual mCherry positive, control and amotl2 MO aortic endothelial cells, as well as amotl2 MO cells rescued by co-injection with human amotL2 mRNA (control n =18 cells, amotl2 MO n =10 cells, amotl2 MO+ hAMOTL2 mRNA n =11 cells, Ctrl versus amotL2 MO P =0.011, Ctrl versus amotL2 MO+ hamotL2 mRNA P =0.541. ( c ) Quantification of length to height ratio in individual mCherry positive, control and amotl2 MO aortic endothelial cells (Ctrl versus amotL2 MO P =0.0003, Ctrl versus amotL2 MO+ hamotL2 mRNA P =0.722). P -values were calculated by student’s t -test. Error bars indicate s.d. NS, non significant. ( d ) Endothelial actin cytoskeletal structure visualized in the dorsal aortic endothelia from living 48 h.p.f. Tg(cdh5:gal4) mu101 ; Tg(UAS:lifeact-GFP) mu271 transgenic fish. Red boxes indicate magnified areas (right). Arrowheads show actin filaments present in the control, and punctuate actin in the amotl2 MO. Arrows indicate cortical actin present in both control and amotl2 MO embryos. By introducing human amotL2 mRNA, actin filaments could be restored (arrowheads). Scale bar 10 μm. ( e ) In control Tg(fliep:GFF) ubs3 ; (UAS:mRFP); (UAS:VE-cadherinΔC-EGFP) ubs12 embryos (top), where VE-cadherin is tagged to EGFP, and endothelial cells labelled by mRFP, VE-cadherin enmarks cell–cell junctions. In amotL2 MO embryos (bottom), VE-cadherin is still localized in between endothelia at sites of aortic constrictions. Boxed areas are magnified to the right, VE-cadherin–EGFP signal indicated with arrowheads. Scale bar 10 μm. ( f ) The apical-membrane sialomucin podocalyxin (arrowheads) is retained in apical membranes of amotl2 MO DA constrictions. Control Tg(fli1a:EGFP) y1 28 h.p.f. embryos (top) and amotl2 MO (bottom). Boxed areas are magnified below. This is also visualized in the optical transverse section (XZ, right). Scale bar, 10 μm. ( g ) In control Tg(fli1a:EGFP) y1 28 h.p.f. embryos (top), anti-laminin staining is basal (arrowheads) and in amotl2 MO, anti-laminin staining is unaffected (arrowheads, bottom). Scale bar, 10 μm. Full size image AmotL2 regulates cytoskeletal organization Next, we assessed whether the observed deficiency in endothelial cell elongation was due to perturbations in cytoskeletal architecture. In order to study actin reorganization in real time, we used a transgenic fish expressing Lifeact (a 17-amino-acid peptide that binds to filamentous actin) fused to green fluorescent protein (GFP) [35] . Vascular-specific expression of Lifeact-GFP was directed by the VE-cadherin promoter. In control fish, Lifeact signal was mainly localized to cortical junctional actin, as well as to radial actin fibres connecting perpendicularly to endothelial junctions ( Fig. 3d ). Of particular interest, in amotl2 morphant Lifeact fish, these fibres were disrupted and positive signals were detected in intracellular punctae instead ( Fig. 3d ). Lifeact signals associated with cortical actin were not detectably affected in amotl2 morphants ( Fig. 3d ). The actin fibre network could be restored by reintroduction of human amotL2 mRNA ( Fig. 3d ). A similar actin filament defect was observed by phalloidin immunofluorescence staining of zebrafish embryos. ( Supplementary Fig. 2b,c ). Parallel analysis of tnnt2 morphants showed that endothelial cells maintained the cellular shape and the actin filament network also in the absence of circulation ( Supplementary Fig. 3b–e ). We therefore concluded that the amotL2 effect on endothelial morphogenesis was not an indirect effect of perturbed axial circulation. We went on to assess whether the observed cytoskeletal phenotype was associated with defects in mislocalization of junctional proteins. VE-cadherin localization was analysed in live VE-cadherin–EGFP transgenic fish as well as by whole mount immunostaining using VE-cadherin-specific antibodies ( Fig. 3e and Supplementary Fig. 4a ). Both approaches showed junction localization of VE-cadherin even with the altered morphology of the amotl2 morphant aortic endothelial cells. This was also the case with the ZO1 tight junction marker ( Supplementary Fig. 4b ). To assess apical–basal cell polarity in morphant embryos, we also analysed the localization of apical podocalyxin and basement membrane laminin. In amotl2 MO, podocalyxin was observed in a seam-like pattern between paired endothelial cells of the morphant aortae, suggesting that apical polarity had been established and that membrane translocation of podocalyxin was not affected ( Fig. 3f ). Likewise, basement membrane anti-laminin staining was unaffected ( Fig. 3g ). Taken together, the in vivo experiments indicated a specific defect in the actin filaments anchored in the cellular junctions, whereas junction formation and the establishment of apical–basal polarity appeared intact. Inactivation of amotL2 in mouse induces aortic constrictions In order to further understand the role of amotL2, we used a genetic deletion approach to silence gene expression during mouse embryonic blood vessel development. We first examined the expression patterns of amotL2 in vivo, by western blot analysis and whole mount immunofluorescence staining of mouse embryos. A 100 kDa amotL2 band was detected in embryonic lysates from E5 to E19 ( Supplementary Fig. 5a ). Laser scanning confocal microscopy revealed positive amotL2 staining that localized to CD31-positive cellular junctions of the DAe of embryos at E8 ( Fig. 4a ). To inactivate the amotL2 gene in a cell type-specific fashion, we generated mice with loxP sites flanking exon 3 ( Supplementary Fig. 5b ). The resulting amotL2 lox/lox mice were then mated with Cdh5(PAC)-CreERT2 transgenics. The latter allowed efficient tamoxifen-inducible conditional recombinase expression in endothelial cells [36] . Tamoxifen-driven recombination was verified by genomic PCR analysis from embryonic and yolk sac extracts ( Supplementary Fig. 5c ). 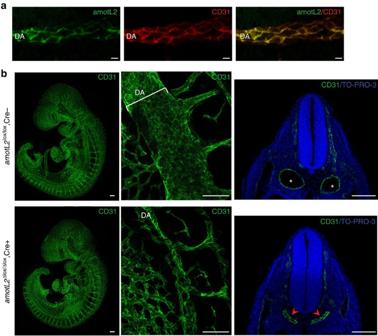Figure 4: Genetic deletion ofAmotl2in mice results in aortic lumen constrictions. (a) amotL2 immunofluorescence staining (green) was detected at cell–cell junctions in aortic endothelial cells of mouse embryos (E8), and colocalized to CD31 staining (red). Scale bar, 10 μm. (b) CD31 staining visualized the blood vessel network of aamotL2lox/lox, Cre−embryo (E9.5). The magnified image (mid panel), showed presence of a DA lumen (bracket marks vessel diameter). The existence of lumens in the paired dorsal aortae was also apparent in the transverse vibratome section (asterisk, 150 μm thickness, right panel). Endothelial cells were labelled with CD31 (green) and TO-PRO-3 was used to visualize nuclei (blue). In somite stagedamotL2Δlox/Δlox, Cre+embryos (E9.5), the general vascular network was present, but in the magnified image (mid panel), it was evident that the lumen of the DA was constricted. This could also be observed in the transverse vibratome section (arrowhead, 150 μm thickness, right panel). Scale bar, 100 μm. Figure 4: Genetic deletion of Amotl2 in mice results in aortic lumen constrictions. ( a ) amotL2 immunofluorescence staining (green) was detected at cell–cell junctions in aortic endothelial cells of mouse embryos (E8), and colocalized to CD31 staining (red). Scale bar, 10 μm. ( b ) CD31 staining visualized the blood vessel network of a amotL2 lox/lox , Cre − embryo (E9.5). The magnified image (mid panel), showed presence of a DA lumen (bracket marks vessel diameter). The existence of lumens in the paired dorsal aortae was also apparent in the transverse vibratome section (asterisk, 150 μm thickness, right panel). Endothelial cells were labelled with CD31 (green) and TO-PRO-3 was used to visualize nuclei (blue). In somite staged amotL2 Δlox/Δlox , Cre + embryos (E9.5), the general vascular network was present, but in the magnified image (mid panel), it was evident that the lumen of the DA was constricted. This could also be observed in the transverse vibratome section (arrowhead, 150 μm thickness, right panel). Scale bar, 100 μm. Full size image At E9.5, amotL2 Δlox/Δlox /Cdh5(PAC)-CreERT2 mice (from here on referred to as amotL2 Δlox/Δlox ) did not differ significantly in size from Cre-negative littermates and were viable ( Fig. 4b ). Analysis of the vascular system of mutants at E9.5 showed that in 80% of mutant embryos, one or both aortae showed lumen defects ( Fig. 5a ). The activity of amotL2 appeared to be dose dependent, as we detected aortic phenotypes in amotL2 heterozygote embryos at similar frequencies ( Fig. 5a ). We also observed aortic constrictions close to the ventricular outflow tract ( Supplementary Fig. 5d ), whereas no defects were detected in littermates that lacked the Cre gene. The efficiency of tamoxifen injections in inducing Cre expression in the vasculature of embryos was monitored in vivo after mating to YFP-reporter mice ( Fig. 5b ). Here, YFP-positive areas (indicating amotl2 recombination) correlated with aortic constrictions ( Fig. 5b ) Similar to our observations in zebrafish, endothelial cells of the aorta in amotL2 -mutant mice exhibited a rounded cell shape ( Fig. 5c ). Other vascular beds such as the lumen of the PCV, ISVs and the brain vascular plexus were not seemingly affected. Furthermore, no detectable inhibition of postnatal retinal angiogenesis could be detected ( Supplementary Fig. 6a,b ). 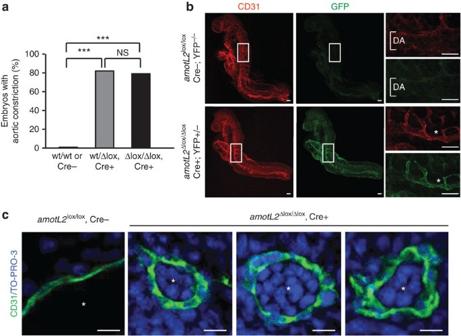Figure 5:amotL2KO induces aortic constrictions and altered endothelial cell shape. (a) Quantification of aortic defects showed presence of aortic constrictions in around 80% of bothamotL2wt/Δlox, Cre+andamotL2Δlox/Δlox, Cre+embryos. All embryos lacking Cre-recombinase expression, as well asamotL2wt/wt, Cre+embryos were considered wt and grouped together.n(amotL2wt/wtor Cre−)=10 embryos, n(amotL2wt/Δlox, Cre+)=11 embryos, n(amotL2Δlox/Δlox, Cre+)=19 embryos). NS, non significant,P-values were calculated by theλ2test. (b) GFP immunofluorescence staining was performed to visualize the YFP reporter, as a marker for Cre-recombinase expression. GFP expression (green) colocalized to CD31 staining (red), in vasculature of E8.5 embryos, arguing for specific expression of GFP in cells expressing CDH5-Cre-recombinase. Constriction of the DA was observed in areas of GFP-positive endothelial cells. Boxed areas are magnified to the right. Aortas of control embryos show a patent lumen (bracket), while inamotL2Δlox/Δloxembryos, the aorta is constricted (asterisk). Scale bar 100 μm. (c) Magnified images from vibratome sections of anamotL2lox/lox, Cre−, as well as three examples ofamotL2Δlox/ΔloxCre+embryos. Images of the latter showed altered shape of aortic endothelial cells, as visualized by CD31 staining (green). Control endothelial cells showed elongated and flat morphology, compared with the short and rounded shape of the endothelial cells from theamotL2Δlox/Δloxembryo. TO-PRO-3 was used for labelling the nuclei (blue). Asterisks indicate DA lumen. Scale bar 10 μm. Figure 5: amotL2 KO induces aortic constrictions and altered endothelial cell shape. ( a ) Quantification of aortic defects showed presence of aortic constrictions in around 80% of both amotL2 wt/Δlox , Cre + and amotL2 Δlox/Δlox , Cre + embryos. All embryos lacking Cre-recombinase expression, as well as amotL2 wt/wt , Cre + embryos were considered wt and grouped together. n ( amotL2 wt/wt or Cre − )=10 embryos, n( amotL2 wt/Δlox , Cre + )=11 embryos, n( amotL2 Δlox/Δlox , Cre + )=19 embryos). NS, non significant, P -values were calculated by the λ 2 test. ( b ) GFP immunofluorescence staining was performed to visualize the YFP reporter, as a marker for Cre-recombinase expression. GFP expression (green) colocalized to CD31 staining (red), in vasculature of E8.5 embryos, arguing for specific expression of GFP in cells expressing CDH5-Cre-recombinase. Constriction of the DA was observed in areas of GFP-positive endothelial cells. Boxed areas are magnified to the right. Aortas of control embryos show a patent lumen (bracket), while in amotL2 Δlox/Δlox embryos, the aorta is constricted (asterisk). Scale bar 100 μm. ( c ) Magnified images from vibratome sections of an amotL2 lox/lox , Cre − , as well as three examples of amotL2 Δlox/Δlox Cre + embryos. Images of the latter showed altered shape of aortic endothelial cells, as visualized by CD31 staining (green). Control endothelial cells showed elongated and flat morphology, compared with the short and rounded shape of the endothelial cells from the amotL2 Δlox/Δlox embryo. TO-PRO-3 was used for labelling the nuclei (blue). Asterisks indicate DA lumen. Scale bar 10 μm. Full size image amotL2 links VE-cadherin to junctional actin filaments In order to gain further insight into how amotL2 might regulate actin architecture, we downregulated amotL2 expression using small interfering RNAs (siRNAs) in cultured mammalian endothelial MS1 cells. amotL2 was located to areas where actin fibres anchor in the VE-cadherin-positive endothelial junctions ( Fig. 6a ). In amotL2 siRNA-treated MS1 cells, VE-cadherin still showed junctional expression, but the connection to actin fibres was lost ( Fig. 6a,b ). Strikingly, amotL2 -depleted cells did not form actin filaments that connect to the cell–cell junctions whereas cortical actin was maintained ( Fig. 6a,b ), consistent with the zebrafish amotl2 MO phenotype ( Fig. 3d ). 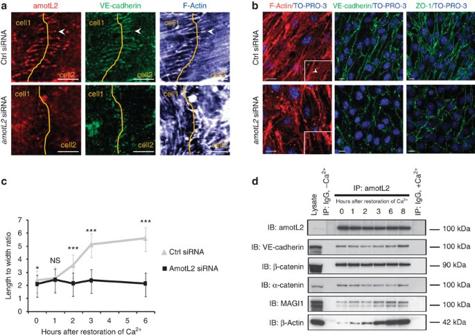Figure 6: AmotL2 is associated with the VE-cadherin–protein complex. (a) Phalloidin staining visualized axial actin fibres (grey) that insert into the anti-VE-cadherin-positive endothelial adherens junctions (green). amotL2 (red) colocalized with actin fibres where they insert into the junction between the apposed endothelial surfaces (arrowheads). Yellow line indicates the cell–cell interface. When amotL2 levels were depleted by siRNA, VE-cadherin was still present at cell–cell junctions, but its connection to actin fibres were lost. (b) In MileSven1 pancreatic islet endothelial (MS1) cells, F-actin fibres were visualized with phalloidin staining (red) (magnified in box to the lower right, arrowhead). Actin fibres were absent inamotL2siRNA-treated cells, but cortical actin belts were still present. The adherens and tight junction-associated proteins, VE-cadherin and ZO-1 (green) were still present at cell–cell contacts inamotL2siRNA-treated MS1 cells. Scale bar, 10 μm. (c) Calcium switch time course experiment showing that reformation of VE-cadherin-based adherens junctions with calcium induces cell elongation as measured by progressively increasing length to width ratio in control siRNA-treated MS1 cells.amotL2siRNA-treated MS1 cells did not elongate even after re-addition of calcium.n>45 cells per group.P(0h)=0.017,P(1h)=0.494,P(2h)=1.443 × 10−13,P(3h)=1.306 × 10−25,P(6h)=1.694 × 10−34.P-values were calculated by the student’st-test. Error bars indicate s.d. NS, nonsignificant. (d) Co-immunoprecipitation of amotL2 followed by western blot analysis at different time points after re-addition of Ca2+. The association of the VE-cadherin/catenin complex to amotL2 was independent of calcium levels. On the contrary, MAGI1 and β-Actin only associated to the VE-cadherin/catenin/amotL2 complex after restoration of calcium levels. Figure 6: AmotL2 is associated with the VE-cadherin–protein complex. ( a ) Phalloidin staining visualized axial actin fibres (grey) that insert into the anti-VE-cadherin-positive endothelial adherens junctions (green). amotL2 (red) colocalized with actin fibres where they insert into the junction between the apposed endothelial surfaces (arrowheads). Yellow line indicates the cell–cell interface. When amotL2 levels were depleted by siRNA, VE-cadherin was still present at cell–cell junctions, but its connection to actin fibres were lost. ( b ) In MileSven1 pancreatic islet endothelial (MS1) cells, F-actin fibres were visualized with phalloidin staining (red) (magnified in box to the lower right, arrowhead). Actin fibres were absent in amotL2 siRNA-treated cells, but cortical actin belts were still present. The adherens and tight junction-associated proteins, VE-cadherin and ZO-1 (green) were still present at cell–cell contacts in amotL2 siRNA-treated MS1 cells. Scale bar, 10 μm. ( c ) Calcium switch time course experiment showing that reformation of VE-cadherin-based adherens junctions with calcium induces cell elongation as measured by progressively increasing length to width ratio in control siRNA-treated MS1 cells. amotL2 siRNA-treated MS1 cells did not elongate even after re-addition of calcium. n >45 cells per group. P (0h)=0.017, P (1h)=0.494, P (2h)=1.443 × 10 −13 , P (3h)=1.306 × 10 −25 , P (6h)=1.694 × 10 −34 . P -values were calculated by the student’s t -test. Error bars indicate s.d. NS, nonsignificant. ( d ) Co-immunoprecipitation of amotL2 followed by western blot analysis at different time points after re-addition of Ca 2+ . The association of the VE-cadherin/catenin complex to amotL2 was independent of calcium levels. On the contrary, MAGI1 and β-Actin only associated to the VE-cadherin/catenin/amotL2 complex after restoration of calcium levels. Full size image The integrity of VE-cadherin-based adherens junctions is calcium dependent and can be modulated by withdrawal and subsequent re-addition of calcium [37] . Re-addition of calcium to calcium-depleted MS1 cells resulted in synchronous cell shape changes correlating with formation of actin filaments associated to endothelial junctions ( Supplementary Fig. 7b ). In contrast, knockdown of amotL2 in MS1 cells rendered the cells refractory to calcium-induced cell shape changes ( Fig. 6c ). In addition, in ctrl siRNA MS1 cells, calcium re-addition caused relocalization of VE-cadherin and amotL2 from the cytoplasm to cell junctions with similar kinetics ( Supplementary Fig. 7b ). We and others have shown that the Amot family of proteins associates to the scaffold junctional protein MAGI1 via a WW protein interaction motif [38] , [39] . It has further been reported that MAGI1 associates to VE-cadherin via binding to β-catenin [40] , [41] . These findings raised the question whether amotL2 functions together with VE-cadherin in controlling cytoskeletal architecture. Therefore, we performed co-immunoprecipitation of amotL2 and associated proteins before and after re-addition of calcium. As shown in Fig. 6d , VE-cadherin, MAGI1, β-catenin, α-catenin and β-actin were pulled down together with amotL2 in MS1 endothelial cells. Of interest, amotL2 association with β-actin correlated with actin fibre formation and cell elongation ( Fig. 6d ). Analysis of the amotL2/VE-cadherin complex We further analysed the biochemical composition of the VE-cadherin/amotL2 complex. To this end, we mutated the putative WW-binding motifs located in the N-terminal domain of amotL2, by exchanging the tyrosine to an alanine ( Fig. 7a ). Co-immunoprecipitation analysis showed that the LPTY but not the PPQY motif was required for the association to MAGI1 and β-actin, while neither of the sites were important for the binding to VE-cadherin or β-catenin ( Fig. 7b ). The importance of the LPTY site was further underscored by functional analysis in zebrafish. mRNA encoding wt, LPTA or PPQA-mutant human amotL2 were co-injected with amotL2 morpholinos into zebrafish embryos as described in previous sections. Mutation of the LPTY motif completely abrogated the rescue effect of the injected mRNA while the PPQA mutant rescued the circulatory phenotype to the same extent as the wild-type mRNA ( Fig. 7c ). As shown in Fig. 7d , MAGI1 could be co-immunoprecipitated together with amotL2 and VE-cadherin. However, the binding of MAGI1 to VE-cadherin was lost in amotL2 siRNA-depleted cells. These data suggested that amotL2 coupled MAGI1 and actin fibres to the VE-cadherin junctional complex. We next used amotL2 deletion constructs (shown in Fig. 7a ) to narrow down the sequences essential for the association with VE-cadherin. Co-immunoprecipitation analysis localized the VE-cadherin and β-catenin binding site to the 101-307a.a. of the N-terminal domain of amotL2 ( Fig. 7e ). 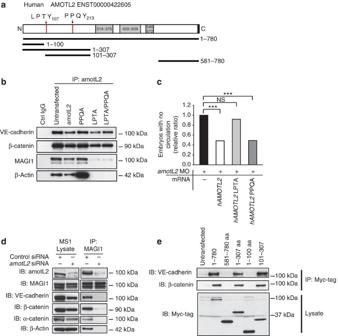Figure 7: AmotL2 association with VE-cadherin controls actin fibre formationin vitro. (a) Schematic model showing the different domains of the human amotL2 protein (ensembl accession code ENST00000422605). Putative coil–coil domains (314–375, 420–509, 545–572), carboxy-terminal PDZ-binding motif and the amino-terminal LPTY (107) and PPQY (213) WW-binding sites. In addition, the different amotL2 deletion constructs used are shown. (b) Endogenous amotL2, as well as the wild-type construct co-immunoprecipitates with VE-cadherin, β-catenin, α-catenin, MAGI1 and β-Actin and in MS1 cells. Mutation of the PPQY motif did not affect the binding to the VE-cadherin adherens junction complex. When the LPTY motif was mutated to LPTA, the binding of amotL2 to MAGI1 and β-Actin was lost. The double mutant (LPTA/PPQA) showed a binding efficiency similar to the LPTA mutation alone. (c) TheamotL2MO circulatory phenotype in 48 h.p.f. zebrafish embryos could be rescued by injection of the wild-type humanamotL2mRNA, and the mRNA with a mutation in the PPQY motif. The LPTA-mutant mRNA did not restore circulation.n(amotL2MO)=215 embryos,n(amotL2MO+ hamotL2mRNA)=193 embryos,n(amotL2MO+ hamotL2LPTA mRNA)=84 embryos,n(amotL2MO+ hamotL2PPQY mRNA)=181 embryos. NS, nonsignifcant.P-values were calculated by theλ2test. (d) When immunoprecipitation was performed after silencing of amotL2 expression by siRNA, MAGI1 association to the VE-cadherin/catenin protein complex was abrogated. In addition, the binding of MAGI1 to β-Actin was lost. (e) Full-length amotL2-Myc (1–780 aa) or the indicated Myc-tagged amotL2 deletion constructs were transfected into MS1 cells. amotL2 was immunoprecipitated from cell lysates using anti-Myc antibody. Only constructs containing the 101–307 aa domain was able to interact with VE-cadherin and β-catenin. Figure 7: AmotL2 association with VE-cadherin controls actin fibre formation in vitro. ( a ) Schematic model showing the different domains of the human amotL2 protein (ensembl accession code ENST00000422605). Putative coil–coil domains (314–375, 420–509, 545–572), carboxy-terminal PDZ-binding motif and the amino-terminal LPTY (107) and PPQY (213) WW-binding sites. In addition, the different amotL2 deletion constructs used are shown. ( b ) Endogenous amotL2, as well as the wild-type construct co-immunoprecipitates with VE-cadherin, β-catenin, α-catenin, MAGI1 and β-Actin and in MS1 cells. Mutation of the PPQY motif did not affect the binding to the VE-cadherin adherens junction complex. When the LPTY motif was mutated to LPTA, the binding of amotL2 to MAGI1 and β-Actin was lost. The double mutant (LPTA/PPQA) showed a binding efficiency similar to the LPTA mutation alone. ( c ) The amotL2 MO circulatory phenotype in 48 h.p.f. zebrafish embryos could be rescued by injection of the wild-type human amotL2 mRNA, and the mRNA with a mutation in the PPQY motif. The LPTA-mutant mRNA did not restore circulation. n ( amotL2 MO)=215 embryos, n ( amotL2 MO+ h amotL2 mRNA)=193 embryos, n ( amotL2 MO+ h amotL2 LPTA mRNA)=84 embryos, n ( amotL2 MO+ h amotL2 PPQY mRNA)=181 embryos. NS, nonsignifcant. P -values were calculated by the λ 2 test. ( d ) When immunoprecipitation was performed after silencing of amotL2 expression by siRNA, MAGI1 association to the VE-cadherin/catenin protein complex was abrogated. In addition, the binding of MAGI1 to β-Actin was lost. ( e ) Full-length amotL2-Myc (1–780 aa) or the indicated Myc-tagged amotL2 deletion constructs were transfected into MS1 cells. amotL2 was immunoprecipitated from cell lysates using anti-Myc antibody. Only constructs containing the 101–307 aa domain was able to interact with VE-cadherin and β-catenin. Full size image amotL2 mediates mechanical force at cellular junctions Our data showed that amotL2 linked VE-cadherin to actin fibres that were coupled perpendicular to cellular junctions. The recent evidence that cadherin–protein complexes are sites of mechanotransduction raised the possibility that amotL2 integrated actomyosin contractile forces, required for lumen expansion [17] . First, we assessed whether chemical inhibition of actin contraction using the non-muscle myosin inhibitor blebbistatin could phenocopy the effect of amotl2 MO in zebrafish. In agreement with amotl2 MO, blebbistatin treatment between 18–20 h.p.f. caused loss of circulation and reduced length to width and length to height ratios in mCherry-labelled dorsal aortic endothelia in vivo and in MS1 cells in vitro ( Fig. 8a–d , Supplementary Fig. 8a,e,f ). Furthermore, actomyosin contractility appeared essential for the maintenance of lumen expansion, as treatment of embryos after initiation of axial vessel circulation induced collapse of the DA ( Supplementary Fig. 8d ). Taken together, these data supported the notion that contractile mechanical forces were required for aortic luminal expansion. 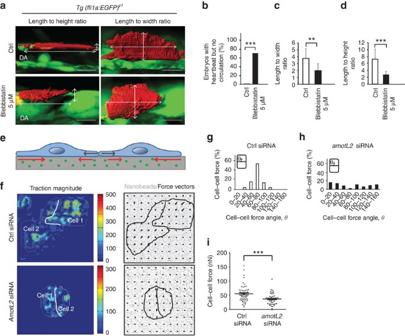Figure 8: AmotL2 is required for generation of actomyosin dependent cell–cell force. (a) Zebrafish embryos treated with 5 μM of the actomyosin-inhibiting drug blebbistatin, during aortic lumen formation (18–20 h.p.f.) show defective circulation at 30 h.p.f. Sagittal (left) and dorsal (right), view of individual mCherry-positive DA endothelial cells in theTg(fli1a:EGFP)y1embryos (30 h.p.f.). Bidirectional arrows indicate the length and width dimensions. In blebbistatin-treated embryos, DA endothelial cells have altered cell shape. Scale bar 10 μm. (b) Quantification of the circulatory phenotype in blebbistatin-treated embryos (n(ctrl)=57 embryos,n(blebbistatin)=121 embryos,P-value calculated by theλ2test). (c) Quantification of length to width ratio in dorsal aortic endothelia from blebbistatin-treated zebrafish embryos (controln=18 cells, blebbistatin treatedn=11 cells,P=1.8 × 10−3). (d) Quantification of length to height ratio in aortic endothelia from blebbistatin-treated zebrafish embryos (P=3.8 × 10−5).P-values calculated by the student’st-test. (e) Illustration of the traction force microscopy experiment. MS1 cell–cell doublets were seeded onto hydrogel-embedded fluorescent beads (green). As the cells produce force, the consequent movement of the beads was used to calculate both the cell traction force (red arrows) and further the cell–cell force (black arrows) with Fourier Transform Traction Cytometry. (f) Traction stress magnitudes of a cell doublet (left). Grey line indicate the outline of the cells and the bold white line the region of the cell–cell junction used to calculate the force imbalance within the cell doublet. Stresses are given in Pascal. The images were divided into 10 × 10 squares and the resultant traction vector of each square was calculated (magnitude and angle) and presented (right, black arrows) superimposed with GFP-tagged nanobeads (200 nm, grey). Black lines indicate cell borders. For original image of traction vectors seeSupplementary Fig. 5h. (g,h) Histogram presenting quantification of the angles between the cell–cell force and the cell–cell contact in the shown cell doublets. Pattern of force angle distribution between ctrl siRNA andamotL2siRNA cell doublets was significantly different. KS=0.35,P=9.29 × 10−5.P-value was calculated by the Kolmogorov–Smirnov test. (i) Scatter plot of the cell–cell force comparing ctrl siRNA-treated MS1 cell doublet (n=54, mean±s.d. is 55±29 nN) andamotL2siRNA-treated MS1 cell doublet (n=45, mean±s.d. is 37±19 nN),P-value was calculated by the student’st-test. Figure 8: AmotL2 is required for generation of actomyosin dependent cell–cell force. ( a ) Zebrafish embryos treated with 5 μM of the actomyosin-inhibiting drug blebbistatin, during aortic lumen formation (18–20 h.p.f.) show defective circulation at 30 h.p.f. Sagittal (left) and dorsal (right), view of individual mCherry-positive DA endothelial cells in the Tg(fli1a:EGFP) y1 embryos (30 h.p.f.). Bidirectional arrows indicate the length and width dimensions. In blebbistatin-treated embryos, DA endothelial cells have altered cell shape. Scale bar 10 μm. ( b ) Quantification of the circulatory phenotype in blebbistatin-treated embryos ( n (ctrl)=57 embryos, n (blebbistatin)=121 embryos, P -value calculated by the λ 2 test). ( c ) Quantification of length to width ratio in dorsal aortic endothelia from blebbistatin-treated zebrafish embryos (control n =18 cells, blebbistatin treated n =11 cells, P =1.8 × 10 −3 ). ( d ) Quantification of length to height ratio in aortic endothelia from blebbistatin-treated zebrafish embryos ( P =3.8 × 10 −5 ). P -values calculated by the student’s t -test. ( e ) Illustration of the traction force microscopy experiment. MS1 cell–cell doublets were seeded onto hydrogel-embedded fluorescent beads (green). As the cells produce force, the consequent movement of the beads was used to calculate both the cell traction force (red arrows) and further the cell–cell force (black arrows) with Fourier Transform Traction Cytometry. ( f ) Traction stress magnitudes of a cell doublet (left). Grey line indicate the outline of the cells and the bold white line the region of the cell–cell junction used to calculate the force imbalance within the cell doublet. Stresses are given in Pascal. The images were divided into 10 × 10 squares and the resultant traction vector of each square was calculated (magnitude and angle) and presented (right, black arrows) superimposed with GFP-tagged nanobeads (200 nm, grey). Black lines indicate cell borders. For original image of traction vectors see Supplementary Fig. 5h . ( g , h ) Histogram presenting quantification of the angles between the cell–cell force and the cell–cell contact in the shown cell doublets. Pattern of force angle distribution between ctrl siRNA and amotL2 siRNA cell doublets was significantly different. KS=0.35, P =9.29 × 10 −5 . P -value was calculated by the Kolmogorov–Smirnov test. ( i ) Scatter plot of the cell–cell force comparing ctrl siRNA-treated MS1 cell doublet ( n =54, mean±s.d. is 55±29 nN) and amotL2 siRNA-treated MS1 cell doublet ( n =45, mean±s.d. is 37±19 nN), P -value was calculated by the student’s t -test. Full size image The striking effect of amotL2 depletion on the junctional actin filament organization suggested a role in mediating the mechanical load on cellular adhesions. To test this hypothesis, we employed traction force microscopy to measure tension between pairs of endothelial cells. This method has been described by Gardel and coworkers [19] and the junctional force is indirectly calculated by measuring forces exerted on the extracellular matrix [42] . Control or amotL2 siRNA-depleted MS1 cells were plated on fibronectin, which had been chemically cross-linked to polyacrylamide gels. Forces applied on the cell–extracellular matrix interface were quantified by measuring the displacement of fluorescent beads before and after removal of cells by trypsinization. The force transmitted between doublets of cells was determined using a calculation of the imbalance of traction forces exerted on the focal adhesions ( Fig. 8e,f ) [19] . The net force exercised on the junctions was significantly lower in the amotL2-depleted cells ( Fig. 8f,i ). In addition, in control cells, forces were directed perpendicular to the cell junctions, whereas the directional force was lost in the amotL2 siRNA-treated cells ( Fig. 8g,h ). A schematic is shown in Fig. 9a showing how force is transmitted via endothelial adherent junctions through the VE-cadherin/amotL2 complex leading to the expansion of the aortic lumen ( Fig. 9b ). 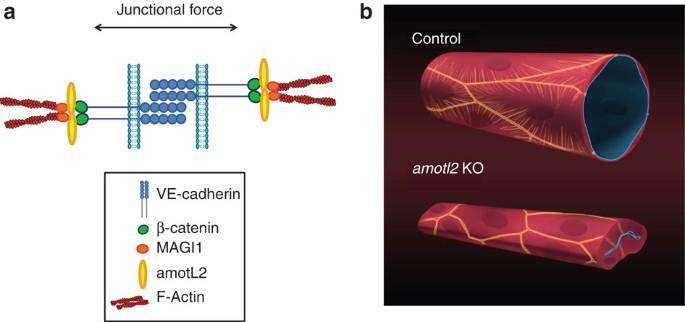Figure 9: Proposed model of the function of the VE-cadherin/AmotL2 complex during aortic lumen expansion. (a) AmotL2 is needed for the connection of the VE-cadherin/catenin complex to MAGI1 and actin filaments, and for transmission of force between neighbouring cells via the cellular junctions. (b) amotL2 knockdown results in perturbed lumen expansion or collapse of the DA. The DA is made of elongated and flat endothelial cells that are connected by actin fibres (shown as yellow spikes). Actin fibres insert into the apposing endothelial adherens junctions (yellow borders), and enables transcellular transmission of mechanical force, and thus endothelial elongation. InamotL2KD animals, polarized endothelia (apical membranes are shown in blue) lack radial actin fibres, resulting in failed cell morphogenesis and luminal constrictions. Figure 9: Proposed model of the function of the VE-cadherin/AmotL2 complex during aortic lumen expansion. ( a ) AmotL2 is needed for the connection of the VE-cadherin/catenin complex to MAGI1 and actin filaments, and for transmission of force between neighbouring cells via the cellular junctions. ( b ) amotL2 knockdown results in perturbed lumen expansion or collapse of the DA. The DA is made of elongated and flat endothelial cells that are connected by actin fibres (shown as yellow spikes). Actin fibres insert into the apposing endothelial adherens junctions (yellow borders), and enables transcellular transmission of mechanical force, and thus endothelial elongation. In amotL2 KD animals, polarized endothelia (apical membranes are shown in blue) lack radial actin fibres, resulting in failed cell morphogenesis and luminal constrictions. Full size image A major issue in the vascular development is how individual endothelial cells collectively unite in the formation of tubes. How do endothelia interpret, integrate and translate multiple cues into defined, reproducible cytoskeletal architectures and multicellular organization structures? In this report, we provide mechanistic insight into how mechanical force via cell–cell adhesions and the cytoskeletal network coordinate aortic lumen expansion. This process involves the protein amotL2 that links the generation of VE-cadherin-associated contractile actin filaments to cell and tissue morphogenesis. Endothelial cells elongate in the anterior–posterior axis during aorta formation. In our studies, we could show that this cellular shape change was not dependent on the shear stress exerted by blood flow. Instead, we propose that endothelial morphogenesis during aortic lumen formation is dependent on the tensile forces exerted via the VE-cadherin/amotL2 junctional complex. This notion was supported by our findings that short-term treatment with the myosin inhibitor blebbistatin mimicked the effects of amotL2 depletion. In addition, we could show that amotL2 was essential for the transmission of junctional force between endothelial cells in vitro . This finding is significant, as it shows how amotL2 enables the formation of transcellular actin cables that share mechanical actin and tension in between cells. Further, this allows lumen expansion to become a collective event that is needed for the synchronization with the onset of circulation. It was apparent that amotL2 inactivation specifically affected aortic function, whereas the vein lumen formation appeared to be intact. The mechanisms of how these two tubular structures are formed may provide an explanation for this. Similar to epithelial lumen formation in vitro , the aortic lumen is generated between adjacent endothelial cells by establishment of apical–basal polarity and the subsequent repulsion and expansion requires accumulation of fluid pressure and actin contraction. There are other principles described for the development of large calibre vessels such as the common cardinal vein. Here, lumen is formed by ensheathment of preexisting luminal space [35] . Inherent differences in the mechanisms of lumen formation may therefore explain why amotL2 is essential for aortic and not vein lumen formation. We did notice a slight delay in ISV formation in amotL2 MO embryos; however, no detectable difference was observed compared with control embryos at 48 h.p.f. Furthermore, inactivation of amotL2 during postnatal retinal angiogenesis did not affect endothelial cell migration. An indirect effect on ISV formation, due to defects in the DA, may therefore explain the apparent discrepancies between our data and what has previously been reported [43] . VE-cadherin has previously been shown to be essential for multiple biological processes that influence endothelial cells, such as proliferation, migration, permeability and polarity [44] . Our data show that amotL2 is a downstream effector of VE-cadherin controlling cell elongation and junctional force. We propose a model, whereby amotL2 integrates VE-cadherin junctional signalling to endothelial actin fibre assembly during DA lumen expansion ( Fig. 9 ). This may occur in conjunction with other cellular mechanisms for lumen expansion, like electrostatic repulsion and vectoral fluid transport [45] , [46] . Taken together, we have identified a novel mechanism by which force can be transmitted across cells via adherens junctions and actin fibres. Further studies may show whether the connection between amotL2, adherens junctions, and the actin network is a unifying principle in lumen formation in tubular epithelial and ductal organs. Mouse experiments Animal experiments were performed according to a permit from the Stockholm South ethical committee in Sweden. The amotL2 conditional knockout mice were crossed with Cdh5(PAC)–CreERT2 as well as ROSA26–EYFP reporter mice. All the animals were in C57BL/6 background. Mouse tail tips, yolk sacs or embryos were used for genotyping. The primers used in genomic PCR are as follows: for amotL2 flox gene: 5′-CTAGGAGCACGTGGAAGACC-3′ (forward)5′-GGGCTAGCTGCTCTACAAGG-3′ (reversed); for amotL2 deflox gene: 5′-CAGGAGGATCACACCACCAG-3′ (forward)5′-CAGCAAG TGGAAAGCCTGAG-3′ (reversed). To investigate the function of amotL2 during mouse embryonic development, tamoxifen was intraperitoneally injected into pregnant amotL2 lox/lox /Cdh5(PAC)–CreERT2/ROSA26–EYFP mice from E5.5 to E8.5. The dose of tamoxifen was 0.5 mg for E5.5 and 1.0 mg per day for the remaining 3 days. Embryos were collected at E9.5 and fixed with 4% paraformaldehyde (PFA). To analyse the function of amotL2 during postnatal retina angiogenesis, intragastric injection with tamoxifen (50 μg per day from P1 to P3) was performed on amotL2 lox/lox /Cdh5(PAC)–CreERT2/ROSA26–EYFP male and female pups [47] . Mouse retinas were dissected at P6 and fixed with PFA for immunostaining. Zebrafish Zebrafish were raised and maintained according to the standard protocols and in accordance with the regulations set out by the Swedish Board of Agriculture for the use of laboratory animals in scientific research. The following transgenic lines were used in this study: Tg(kdrl:EGFP) s843 (ref. 34 ); Tg(gata1:dsRed) sd2 (ref. 48 ); Tg(fli1a:EGFP) y1 (ref. 49 ); Tg(kdrl:msna-EGFP) is1 (ref. 50 ); Tg(cdh5:gal4) mu101 (ref. 51 ); Tg(UAS:lifeact-GFP) mu271 ; Tg(fliep:GFF) ubs3 ; Tg(UAS:mRFP) ; Tg(UAS:VE-cadherinΔC-EGFP) ubs12 [52] (ref. 52). For vascular-specific expression of lifeact-GFP double transgenic embryos Tg(cdh5:gal4) mu101 ; Tg(UAS:lifeact-GFP) mu271 were used, which we refer to in the text as Lifeact fish [35] . Expression analysis Paralogue-specific epitopes were chosen for the production of anti-amotL2a antibodies. Affinity-purified rabbit polyclonal antibodies against the zebrafish amotL2a protein were made using the antibody production services of Innovagen (Lund, Sweden). For amotL2a, antibodies were made against the C-terminal epitope NH2- CQKAPSAVDLFKGVDDVSAE-COOH. Total RNAs were isolated by RNeasy Kit (Qiagen), according to the manufacturer’s instructions. Each sample was reverse-transcribed into cDNA by miScript RT Kit (Qiagen) and was subjected to quantitative real time (qRT)–PCR analysis with miScript SYBR Green PCR Kit (Qiagen). The following oligonucleotides were used: amotl2a f1 5′-GGGCACTTTATGCTCAACTCTTG-3′ amotl2a r1 5′-CGGCCTTGCTCTCGTCTT-3′ amotl2b f1 5′-CGCCCTTCAGCGAAGTTATTC-3′ amotl2b r1 5′-CCCGCACAACGTGACAATG-3′ Mouse amotL2 was detected with a rabbit affinity-purified antibody made against the C-terminal motif of human amotL2 (Innovagen, Lund, Sweden); NH2-CLDSVATSRVQDLSDMVEILI-COOH. Western blotting Dechorionated zebrafish embryos were mechanically homogenized in SDS sample buffer, after removal of the yolk, and loaded onto 10% Bis-Tris gel. Cells were lysed with Triton X-100 before samples were loaded onto the gel. The following antibodies were used: anti-VE-cadherin (1:500, #555289, 11D4.1, BD Biosciences), anti-β-catenin (1:500, #610154, 14/beta-catenin, BD Biosciences), anti-α-catenin (1:500, #610193, 5/alpha-catenin, BD Biosciences), anti-MAGI1 (1:500, #WH0009223M3, 7B4, Sigma), anti-β-actin (1:20000, #ab3280, ALTN05CC4, Abcam). The mouse embryo E5-E19 western blot was ordered from Zyagen and amotL2 was detected with a rabbit affinity-purified antibody against the C-terminal motif of human amotL2; NH2-CLDSVATSRVQDLSDMVEILI-COOH (1:500). Uncropped scans of the western blots are provided as Supplementary Figs 9–12 . Cloning of zebrafish amotl2a and amotl2b genes Database searches on Ensembl and NCBI with hAMOTL2 identified two amotl2 orthologues in the zebrafish genome. The sequence of amotl2a has previously been published [32] . To verify the putative amotl2b sequence, the complete gene was cloned and sequenced from a cDNA zebrafish library isolated from 48 h.p.f. embryos. amotl2a sequences were cloned by real-time PCR using the following primers and TOPO cloned into pCRII (Invitrogen) using the following primers: amotl2a forward 5′-ATGAGAACGGCAGAGGAATC-3′ amotl2a reverse 5′-TGGACATTGTTATCTCAGATG-3′ amotl2b f1 5′-ACCAGGTGGACTACCAGCA-3′ amotl2b r1 5′-GTTCCTGCTCTAGCCGTGTC-3′ amotl2b f2 5′-GGAGAAGGCCCTCAAAATTC-3′ amotl2b r2 5′-AGCTCCGTTATTGAGCTGGA-3′ Morpholino knockdown experiments Morpholinos were purchased from Gene Tools (Philomath, Oregon, USA). The following morpholinos were used in this study: amotl2a MO 5′-CTGATGATTCCTCTGCCGTTCTCAT-3′ amotl2b MO1 5′-TGAGTATTTATGATCTGAGCTGAAC-3′ amotl2b MO2 5′-TGAGTATTTATGATCTGAGCTGAAC-3′ amotl2b MO3 5′-AGCTGAGTCAGTGTACCTTCTGAAT-3′ tnnt2 5′-CATGTTTGCTCTGATCTGACACGCA-3′ control 5′-CCTCTTACCTCAGTTACAATTTATA-3′ The tnnt2 morpholino has been published [33] . The amotl2a morpholino was injected at 1.25 ng per embryo and the amotl2b morpholino was injected at 2.5 ng per embryo. Morpholino-injected zebrafish embryos were maintained at 28 °C in standard E3 water supplemented with 0.003% phenyl-2-thiourea. Gene knockdown was confirmed molecularly by RT–PCR ( amotl2b ) or western blot ( amotl2a ). Circulation phenotypes were assessed at 48 h.p.f. An mRNA encoding human AMOTL2 or amotL2 mutants were synthesized using the SP6 Message Machine kit (Ambion, Austin, TX, USA), and 50 pg per embryo were co-injected together with the morpholinos. For imaging individual endothelial cells, the Tol2 construct pDEST ( fli1 :mCherryCAAX) was co-injected with Tol2 mRNA into newly fertilized embryos and DA cells were imaged at 28 h.p.f. following standard protocols [53] . Briefly, the vector pDEST ( fli1 :mCherryCAAX) containing Tol2 transposon sequences was co-injected (25 ng μl −1 ) with Tol2 mRNA (35 ng μl −1 ). The Tol2 mRNA was produced by in vitro transcription using mMessage mMachine Kit SP6 (#1340, Ambion). The mixture was injected into one-cell-stage embryos. At 28 h.p.f. embryos were dechorinated and mounted in 1% low-melt agarose on a coverslip for imaging of mCherry-expressing DA cells. Pharmacological experiments Pharmacological experiments with 10 μM cytochalasin D or 50 μM ROCK inhibitor Y-27632 (Sigma) were used to inhibit F-actin polymerization in zebrafish embryos from 18–28 h.p.f. For blebbistatin experiments, zebrafish embryos were treated with 5 μM blebbistatin from 18–20 h.p.f. and then moved to drug-free egg water for recovery. MS1 (Mile Sven1 pancreatic endothelial cells, ATCC CRL-2279) were treated with 5 μM blebbistatin for 2 h, whereupon they were washed with fresh medium. siRNA transfection For siRNA transfections, cells were seeded the day before transfection on glass slides (BD Falcon Cultureslides BD Biosciences) coated with 1% BD Matrigel Basement Membrane Matrix (BD Biosciences) in growth medium without antibiotics. Just before transfection, growth medium was exchanged for OPTI-MEM I Reduced Serum Media (Invitrogen). Smartpool siGENOME siRNAs (Dharmacon/Thermo Scientific) against amotL2 (M-062016-01), as well as non-targeting siRNA Pool #2 (D-001206-14) were transfected into the cells with Oligofectamine Transfection Reagent (Invitrogen) according to the manufacturer’s protocol. siRNAs were used at the final concentrations of 0.32 μM for both control and amotL2 siRNAs. Four hours after transfection serum was added to a final concentration of 20%. Cells were allowed to grow for 72 h prior to the evaluation by immunofluorescence staining or western blot. Cytoo chip experiments Control and amotL2 siRNA-treated MS1 cells were seeded on starter fibronectin-coated Cytoo chips (10-900-10-26, France) and allowed to grow for 3 h. Cells were then fixed in 4% PFA and stained with anti-paxillin and phalloidin (TexasRed-X Phalloidin # T7471, Invitrogen). Calcium switch assay 30,000 cells per well were seeded onto glass slides (BD Falcon Cultureslides BD Biosciences) coated with 1.5% gelatin. Cells were allowed to attach and spread over night. The following day transfection with control and amotL2 siRNA was performed, as described previously. Two days after transfection, medium was changed to calcium-free medium. Twenty-two hours later cells were put back into normal growth medium ( t =0h), and allowed to grow for another 1, 2, 3 and 6 h respectively before fixation. Immunofluorescence staining Cells were washed in phosphate-buffered saline (PBS) and fixed in 4% PFA for 10 min at room temperature (RT). After washing in PBS, permeabilization was performed with 0.1% Triton X-100 for one minute at RT. Cells were again washed in PBS and blocked for 1 h in 5% horse serum (HS) at RT. Antibodies were diluted in the blocking solution, and all incubations were performed at RT. Incubations were 1 h for primary antibodies and 45 min for secondary antibodies. The following antibodies and stains were used; anti-VE-cadherin (1:100, #555289, 11D4.1, BD Biosciences), anti-ZO-1 (1:200, #339100, ZO1-1A12, Invitrogen), anti-paxillin (1:100, #610620, 165/Paxillin, BD Biosciences), anti-laminin (1:200, #L9393, polyclonal, Sigma), TO-PRO-3 iodide (642/661) (1:1000, #T3605, Invitrogen) and phalloidin (1:200, TexasRed-X Phalloidin # T7471, Invitrogen)/Phalloidin-Atto647N (1:200, #65906, Sigma), AlexaFlour 488/568 secondary antibodies (1:1000, Invitrogen). Zebrafish embryos were fixed in 4% PFA/PBS at 4 °C overnight and processed for whole mount immunofluorescence staining following standard protocols. Rabbit antibodies against zebrafish podocalyxin and VE-cadherin/Cdh-5 have been previously published [54] , [55] . For anti-VE-cadherin staining, embryos were fixed in 2% PFA/PBS/0.1% Tween20. Alternatively, 48 h.p.f. Tg(fli1a:EGFP) y1 zebrafish embryos were fixed, sectioned on a Leica Vibratome in 4% low-melt agarose at a thickness of 200 μm. Sections were stained with TexasRed-X Phalloidin for visualizing F-actin and TO-PRO-3 iodide for labelling the nuclei. Images were taken on a Zeiss LSM700 Confocal/Zeiss LSM5 Exciter confocal microscope and processed using ImageJ. Images of endothelial cells expressing mCherryCAAX under the fli1a promoter were processed with Imaris (Bitplane) to create a three-dimensional surface. Images of phalloidin and podocalyxin staining of Tg(fli1a:EGFP) y1 embryos were processed with Imaris (Bitplane) to minimize non-endothelial signal. This was performed by creating a new co-localization channel, showing only the podocalyxin positive pixels that also are positive for EGFP. Mouse embryos (E8 or E9.5) were fixed in 4% PFA at +4 °C, overnight (O/N). Next day embryos were washed with PBS and permeabilized with 0.2% Triton X-100 in PBS at RT. Blocking was performed in 5% HS/0.1% Triton X-100/PBS at +4 °C, O/N. Embryos were washed with 5% HS/0.1% Tween20/PBS before incubation with primary antibody in the same buffer at +4 °C, O/N. After the antibody incubation, embryos were washed first with 5%HS/0.1%Tween20/PBS at +4 °C, and second with 0.1% Tween20 at +4 °C. After washing, embryos were exposed to a second fixation in 4%PFA for one hour at +4 °C. Thereafter, another washing was performed in 0.1%Tween20 in PBS. Secondary antibody incubation was performed as for the primary antibody. On the last day, embryos were washed in 0.1%Tween20 in PBS at +4 °C, fixed again in 4%PFA for 1 hat +4 °C, and washed in 0.1%Tween20 in PBS at +4 °C. Embryos were mounted on coverslips with ProLong Gold anti-fade reagent (#P36930, Invitrogen). For visualization of blood vessels anti-CD31 (#550274, MEC13.3, BD Biosciences) and for confirmation of knock down anti-GFP (#ab6673, polyclonal, Abcam) antibodies were used. For amotL2 staining in mouse aorta, embryos were first sectioned sagittally with a Leica Vibratome in 4% low-melt agarose at a thickness of 350 μm; thereafter, staining and mounting was performed as described above. Co-Immunoprecipitation MS1 endothelial cell lysate were immunoprecipitated with anti-amotL2 polyclonal antibodies (reactive to human amotL2 C-terminal peptide, LDSVATSRVQDLSDMVEILI) or anti-Myc Tag (#05-724, 4A6, Millipore). Immunocomplexes bound to protein A Sepharose beads were gently washed five times with lysis buffer (50 mM HEPES buffer, pH 7.4, 150 mM NaCl, 0.1% SDS, 1% Triton X-100, 1 mM EGTA and protease inhibitors) and separated by SDS-PAGE. amotL2 binding proteins were detected by western blot. Traction force microscopy Polyacrylamide gels were prepared as previously described [56] . Briefly, an acrylamide solution containing 6.67% acrylamide and 0.167% bisacrylamide was mixed with fluorescent beads by sonication before the addition of APS and TEMED. For imaging, an Eclipse T i inverted microscope (Nikon) with a × 60 oil immersion objective (Nikon 60 × 1.4 NA) and a Neo sCMOS camera (Andor Technology) was used. Two images of the beads, before and after cell doublet detachment, and one bright field image of the cell doublet were recorded. The global shift between the beads was determined by cross-correlation of the images. Cell detachment was performed with trypsin (Gibco). The method used for force calculations on continuous substrates was described previously [57] . Briefly, the force exerted by cell1 on cell2 is given by: A similar expression is used to obtain the force exerted by cell2 on cell1. These two forces should be opposite with the same magnitude (the discrepancy between them is used as an estimation of the error on the cell–cell force value). The average tension at the cell–cell interface is estimated by: The fluorescent beads were tracked to obtain a displacement field with high spatial resolution. Using a combination of particle imaging velocimetry and particle tracking, the final displacement field is obtained on a regular grid using linear interpolation. Forces were reconstructed using Fourier transform traction cytometry with zeroth-order regularization, and the cell contractile strength could be estimated by calculating the strain energy U (forces multiplied by displacements), which represents the total energy transferred from the cell to the elastic distortion of the substrate. The force transmitted at a single cell–cell contact between doublets of cells was determined by calculating the balance of traction forces exerted on the extracellular matrix as previously introduced [19] . All calculations and image processing were performed in Matlab. For clearer visibility of force vectors, the images were divided into 10 × 10 squares with a grid. The resultant vector (magnitude and angle) of each square was calculated and presented in Fig. 7 (Original force vectors are shown in Supplementary Fig. 5 ). Statistical analysis For zebrafish experiments, over 60 larvae were analysed per condition. This gave 80% power to detect a 20% difference with 95% confidence. For mouse experiments, 10 embryos were assigned per group. This sample size gave 80% power to detect a 50% phenotypic difference with 95% confidence. For categorical qualitative analysis λ 2 test was used and for quantitative data evaluation two-tailed student’s t -test was performed. Pattern distribution was analysed with Kolmogorov–Smirnov test. How to cite this article: Hultin, S. et al. amotL2 links VE-cadherin to contractile actin fibres necessary for aortic lumen expansion. Nat. Commun. 5:3743 doi: 10.1038/ncomms4743 (2014).